Inverse barocaloric effect in the giant magnetocaloric La–Fe–Si–Co compound Application of hydrostatic pressure under adiabatic conditions causes a change in temperature in any substance. This effect is known as the barocaloric effect and the vast majority of materials heat up when adiabatically squeezed, and they cool down when pressure is released (conventional barocaloric effect). There are, however, materials exhibiting an inverse barocaloric effect: they cool when pressure is applied, and they warm when it is released. Materials exhibiting the inverse barocaloric effect are rather uncommon. Here we report an inverse barocaloric effect in the intermetallic compound La-Fe-Co-Si, which is one of the most promising candidates for magnetic refrigeration through its giant magnetocaloric effect. We have found that application of a pressure of only 1 kbar causes a temperature change of about 1.5 K. This value is larger than the magnetocaloric effect in this compound for magnetic fields that are available with permanent magnets. The need for environmentally friendly cooling technologies has boosted research in solid-state refrigerant materials. In most cases, refrigeration relies on the temperature change caused by the adiabatic application (or removal) of an external field (caloric effects). Under normal circumstances, temperature changes are small, but when the material is close to a phase transition, moderate variations in the external field can provoke temperature changes of several degrees and give rise to so-called giant caloric effects. The tuning parameter for the caloric effect (external field) can be any generalized thermodynamic force, provided that the change in the conjugated generalized thermodynamic displacement is large enough. Hence, giant caloric effects have already been reported for magnetic field (magnetocaloric effect) [1] , [2] , [3] , electric field (electrocaloric effect) [4] , [5] , uniaxial stress (elastocaloric effect) [6] and hydrostatic pressure (barocaloric effect) [7] , [8] . In a recent work [7] , we postulated that most giant magnetocaloric materials would also exhibit large barocaloric effects. This claim is also supported by recent theoretical studies [9] , [10] . Here we report on the barocaloric effect of the giant magnetocaloric material LaFe 11.33 Co 0.47 Si 1.2 . La(Fe,Si) 13 , and the derived quaternary compounds are considered nowadays to be the most promising working materials for magnetic refrigeration technology [11] , [12] . They feature relatively large entropy changes with a very low hysteresis and do not contain toxic materials. Materials with reduced hysteresis are highly desirable because irreversibilites associated with such a hysteresis cause a reduction in the refrigerant capacity [13] , [14] . LaFe 13− x Si x compounds are stable with the cubic NaZn 13 structure (space group ) in a concentration range 1.2 ≤ x ≤ 2.5 (ref. 15 ). Below the Curie temperature T C in the range 200–260 K, the compound orders ferromagnetically, and above T C an itinerant-electron metamagnetic transition is induced by an external field [16] . Such an itinerant-electron metamagnetic transition originates from a magnetic-field-induced change in the density of states of the 3d electrons at the Fermi level [17] . A strong magnetovolume effect originates from the existence of a peak in the electronic density of states, close to the Fermi level, that yields a negative contribution from spin fluctuations to the magnetostriction, resulting in a volume increase on cooling from the paramagnetic to the ferromagnetic state. Two alternative methods have been reported to bring the transition temperature to values close to room temperature without significant modification in the magnetocaloric properties [11] . One method is to add interstitial hydrogen that expands the crystalline lattice and modifies the exchange interaction between iron atoms. Another method is to replace some Fe atoms by other magnetic transition metals. It has been found that replacing Fe by only a few percent of Co enables a fine tuning of the critical temperature, and it has already been possible to produce industrially meaningful quantities (kilograms) of La–Fe–Co–Si material with good magnetocaloric properties around room temperature [18] . The paramagnetic to ferromagnetic transition in La–Fe–Si (and Co-doped) compounds is accompanied by a sizeable volume change of about 1% (ref. 19 ). There is no change in the crystal symmetry, but the sample isotropically expands as it transforms from the high-temperature paramagnetic to the low-temperature ferromagnetic phase. Such a volume change makes the compound highly sensitive to the application of an external hydrostatic pressure; and indeed the effect of pressure on the magnetic and magnetocaloric properties has been reported [16] , [20] . The volume change reported for La–Fe–Si is one of the largest for magnetocaloric materials undergoing magnetostructural transitions. Therefore, this compound is an excellent candidate for exhibiting large barocaloric effects associated with its magnetostructural transition. We have used calorimetry under hydrostatic pressure to obtain the pressure-induced entropy change, and direct temperature measurements to obtain the adiabatic temperature change. These are the two key parameters characterizing a caloric effect. The results are complemented by the measurement of the magnetic field-induced temperature and entropy changes associated with the magnetocaloric effect. The giant barocaloric effect for the material is inverse: that is, we find that the sample warms when pressure is adiabatically released (the entropy decreases under isothermal conditions). The magnetocaloric effect is conventional (the sample warms up when magnetic field is applied and cools down when it is removed). Structural and magnetic characterization The sample studied in this investigation is a polycrystalline LaFe 11.33 Co 0.47 Si 1.2 alloy. X-ray diffraction data (inset in Fig. 1 ) confirm that at room temperature the alloy crystallizes in the NaZn 13 structure (space group ) with a lattice parameter of 11.48 Å. 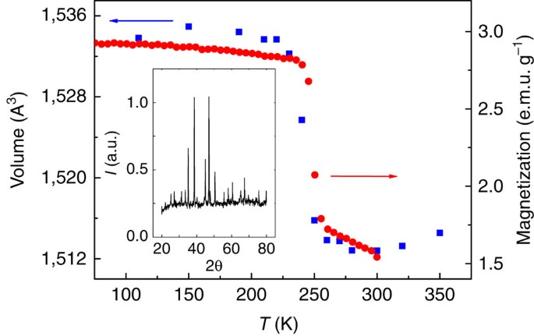Figure 1: Temperature dependence of the volume and the magnetization in LaFe11.33Co0.47Si1.2. Unit cell volume (squares) and low-field magnetization (circles) as a function of temperature. Inset: room temperature X-ray diffraction pattern. The peak at ~45° corresponds toα-iron. When cooled in the absence of an external field, the sample orders ferromagnetically below a temperature T C ~250 K with a concomitant isotropic expansion in the unit cell volume of about 1%, as illustrated in Figure 1 . The most widely used method to compute the entropy change associated with a field-induced caloric effect is from isothermal measurements of the generalized displacement vs force curves. Although this method turns out to be very convenient for determining the magnetocaloric effect, where the magnetization can be measured to high precision using superconducting quantum interference device magnetometry, the method is not readily applicable for determining the barocaloric effect because the involved volume changes are small, and they cannot be measured easily with enough precision. An alternative method is to measure directly the heat exchanged when the transition is thermally induced under an external constant field. It requires the use of purpose-built calorimetric devices, and it has been shown to provide reliable results for various caloric effects. Figure 1: Temperature dependence of the volume and the magnetization in LaFe 11.33 Co 0.47 Si 1.2 . Unit cell volume (squares) and low-field magnetization (circles) as a function of temperature. Inset: room temperature X-ray diffraction pattern. The peak at ~45° corresponds to α -iron. 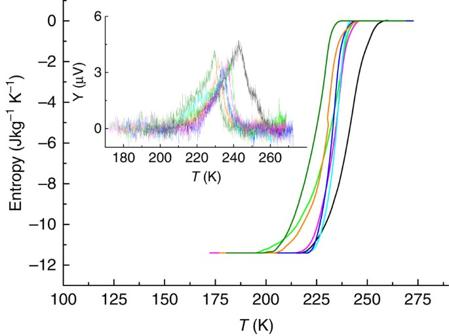Figure 2: Entropy as a function of temperature in LaFe11.33Co0.47Si1.2. Entropy values, referred to the value at ambient temperature, for selected values of hydrostatic pressure. The inset shows calorimetric curves at selected values of the hydrostatic pressure. Curves appear noisy owing to the weakness of the detected signal, associated with the small mass of the sample. Black lines correspond to 0 kbar; green, 0.8 kbar; magenta, 1 kbar; cyan, 1.2 kbar; blue, 1.4 kbar; orange, 1.7 kbar and olive, 2.1 kbar. Full size image Caloric effects Examples of calorimetric curves at selected values of hydrostatic pressure are shown in the inset of Figure 2 . The curves correspond to heating runs, and have been corrected for the baseline drift. An endothermic feature associated with the ferromagnetic–paramagnetic transition is clearly observed. The transition shifts towards lower temperatures as the pressure is increased. This is consistent with pressure enhancing the stability of the lower volume phase, which is the high-temperature phase. The computed entropy changes (integrated entropy curves) at selected values of the hydrostatic pressure are shown in Figure 2 (details of the computation can be found on Methods section). On heating, the entropy increases by 11.4 Jkg −1 K −1 . It must be taken into account that the base-line correction subtracts a background entropy increase, so that the measured increase in entropy is solely due to the occurrence of the phase transition. Numerical subtraction of the integrated entropy curves renders the pressure-induced entropy change (barocaloric effect) at each temperature. 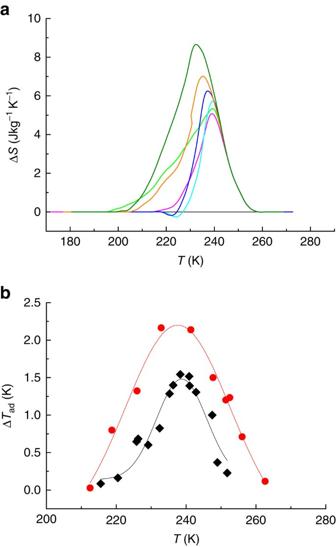Figure 3: Barocaloric effects in LaFe11.33Co0.47Si1.2. (a) Isothermal entropy change as a function of temperature associated with the isothermal application of selected hydrostatic pressures. Black lines correspond to 0 kbar; green, 0.8 kbar; magenta, 1 kbar; cyan, 1.2 kbar; blue, 1.4 kbar; orange, 1.7 kbar and olive, 2.1 kbar. (b)Adiabatic temperature change on fast release of hydrostatic pressure. Diamonds correspond to 1 kbar and circles to 2 kbar (lines are guides to the eye). Results are shown in Figure 3a . The most relevant feature is the positive values of the entropy change, which corresponds to the uncommon inverse barocaloric effect. The magnitude of the barocaloric effect increases with increasing pressures, and a value of 8.6 Jkg −1 K −1 is obtained for p =2095 bar. This value is 75% of the maximum expected value corresponding to the whole transition entropy change. Although the required pressures are larger than typical pressures in domestic fridges (based on compression of a cryogenic gas), they are still readily accessible by conventional hydraulic technologies. Figure 2: Entropy as a function of temperature in LaFe 11.33 Co 0.47 Si 1.2 . Entropy values, referred to the value at ambient temperature, for selected values of hydrostatic pressure. The inset shows calorimetric curves at selected values of the hydrostatic pressure. Curves appear noisy owing to the weakness of the detected signal, associated with the small mass of the sample. Black lines correspond to 0 kbar; green, 0.8 kbar; magenta, 1 kbar; cyan, 1.2 kbar; blue, 1.4 kbar; orange, 1.7 kbar and olive, 2.1 kbar. Full size image Figure 3: Barocaloric effects in LaFe 11.33 Co 0.47 Si 1.2 . ( a ) Isothermal entropy change as a function of temperature associated with the isothermal application of selected hydrostatic pressures. Black lines correspond to 0 kbar; green, 0.8 kbar; magenta, 1 kbar; cyan, 1.2 kbar; blue, 1.4 kbar; orange, 1.7 kbar and olive, 2.1 kbar. ( b )Adiabatic temperature change on fast release of hydrostatic pressure. Diamonds correspond to 1 kbar and circles to 2 kbar (lines are guides to the eye). Full size image In the studied sample, both magnetocaloric and barocaloric effects originate from the same physical mechanism: the strong magnetovolume interplay occuring at the para-ferromagnetic phase transition that encompasses concomitant changes in magnetization and volume. Therefore, it is interesting to compare the barocaloric with the magnetocaloric properties. To this end, we have measured isothermal magnetization curves at selected values of the temperature from which we have numerically computed the entropy change associated with the magnetocaloric effect. The results are consistent with data reported for alloys with compositions close to the studied sample [21] . The magnetocaloric effect is conventional (that is, decrease in entropy on applying a magnetic field), and the magnetic field-induced entropy change at 5 T (−9.2 Jkg −1 K −1 ) amounts to ~80% of the whole transition entropy change. Although entropy change is a good quantity to characterize caloric effects, any practical application requires knowledge of the adiabatic temperature change. Direct measurements of the adiabatic temperature change when pressure is rapidly released are shown in Figure 3b for pressures of 1 and 2 kbar. The first evident result is the confirmation of the inverse character of the barocaloric effect: the sample warms when pressure is released. The temperature dependence of Δ T is in good agreement with that of Δ S ( Fig. 3a ). The adiabatic temperature change can be estimated from isothermal entropy data using , where C is the heat capacity. Although a correct evaluation requires measuring C at different values of p , a rough estimation using C p data measured at atmospheric pressure (inset in Fig. 4 ) shows that the measured values of Δ T are lower than the estimated ones. This difference must be mainly ascribed to a lack of perfect adiabatic conditions in the measurements under pressure due to changes in sample surroundings. Therefore, the actual temperature change is expected to be larger than the data presented in Figure 3b . For comparison we have also directly measured the temperature change associated with the application, Δ T on , and removal, Δ T off , of a magnetic field of 1 T ( Fig. 4 ). The excellent coincidence of |Δ T on | and |Δ T off | is an indication of the negligible irreversible losses for this compound. As a consequence of the good adiabatic conditions in magnetic measurements and low hysteretic losses, the values estimated for Δ T agree fairly well with measured ones. 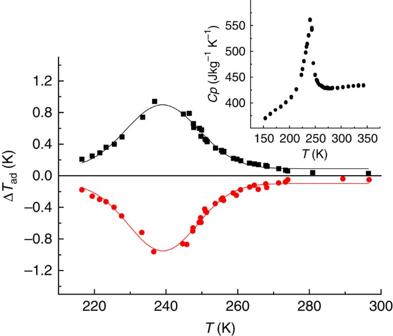Figure 4: Magnetocaloric effect in LaFe11.33Co0.47Si1.2. Adiabatic temperature measurements on applying (ΔTon, squares) and removing (ΔToff, circles) a 1 T magnetic field. Lines are guides to the eye. The inset shows the temperature dependence of the heat capacity at atmospheric pressure and in the absence of magnetic field. Figure 4: Magnetocaloric effect in LaFe 11.33 Co 0.47 Si 1.2 . Adiabatic temperature measurements on applying (Δ T on , squares) and removing (Δ T off , circles) a 1 T magnetic field. Lines are guides to the eye. The inset shows the temperature dependence of the heat capacity at atmospheric pressure and in the absence of magnetic field. Full size image In La–Fe–Si (and doped compounds), the total entropy is due to the magnetic contribution from the itinerant 3 d electrons and a contribution from the lattice (the electronic contribution from the sp conduction electrons is smaller). It has been established that hydrostatic pressure affects both contributions: on the one hand, pressure increases the width of the effective 3 d bands, thus opposing to the onset of the ordered magnetic state. On the other hand, lattice contribution is also affected by pressure through a strong magnetoelastic coupling that modifies phonon frequencies, which can be expressed in terms of a renormalized Debye temperature [9] . In systems undergoing a phase transition involving interplay between different material properties (volume and magnetization in the case of present study), caloric effects associated with each of these properties may be of opposite sign. Actually, in the absence of frustration effects, the primary property providing the dominant change in entropy at the transition should be associated with a conventional caloric effect whereas secondary properties may provide conventional or inverse effects depending on specific features of their coupling to the primary property. For instance, on cooling, Ni–Mn–In magnetic shape-memory alloys undergo a structural transition which involves changes of symmetry and volume and is accompanied by a decrease of the magnetization. Therefore, in this material, the barocaloric effect must be conventional. The decrease in magnetization is a consequence of the interplay of magnetism and structure and originates from the antiferromagnetism associated with the change of distances between Mn atoms induced by the structural transition. This feature explains the well-known inverse magnetocaloric effect in these materials [22] . By contrast, in the La–Fe–Si compounds, the transition is essentially of magnetic nature, and, therefore, the magnetocaloric effect is conventional. Because spin fluctuations induce a volume increase at the transition, the barocaloric effect in this material is inverse. A good parameter to assess the usefulness of a given material for refrigeration purposes is the relative cooling power (RCP) that quantifies the energy absorbed in a refrigerating cycle. A suitable estimation of RCP is provided by the area below the Δ S vs T curve (see Fig. 3a ). The computed values for the magnetocaloric (45 Jkg −1 T −1 ) and barocaloric (90 Jkg −1 kbar −1 ) effects compare well with data for the best giant magnetocaloric materials. Moreover, although magnetic fields stronger than 1 T are difficult to implement, pressures much larger than those used here can be applied (using clamp cells, for instance), and, therefore, the barocaloric effect appears more advantageous because RCP is expected to substantially increase, as a result of a much broader peak resulting from the shift in the transition temperature. In summary, we have identified the occurrence of the barocaloric effect in one of the technologically most promising giant magnetocaloric materials. The barocaloric effect has been found to be inverse, and direct temperature measurements prove that the material heats up on removal of hydrostatic pressure. The magnitude of the barocaloric effect for moderate pressures is larger than the magnetocaloric effect for magnetic fields reachable with permanent magnets, and, therefore, the reported effect is potentially useful for eco-friendly solid-state refrigeration purposes. Finally, it is worth mentioning that the inverse barocaloric effect arises from the volume increase on cooling through the phase transition. Such a volume increase gives rise to a negative thermal expansion (NTE) within a certain temperature range. Materials exhibiting colossal NTE resulting from phase transitions are receiving considerable interest [23] . From thermodynamic arguments, it can be expected that these materials with NTE will also exhibit inverse barocaloric effects. Thermodynamic background For any material subjected to hydrostatic pressure ( p ), magnetic field ( H ) and temperature ( T ) changes, the general expression for an entropy change reads where we have used the Maxwell relations: where β is the thermal expansion. This expression shows that large entropy changes are expected when either volume or magnetization change drastically with temperature under constant external H and p . This situation typically occurs in the vicinity of phase transitions. The sign of the entropy change is determined by the temperature derivatives of M and v . At constant pressure, application of a magnetic field will reduce entropy in those systems for which magnetization decreases with increasing temperature. As this is the most commonly found situation, this effect is termed as conventional magnetocaloric effect. By contrast, in those materials where magnetization increases with increasing temperature, application of a magnetic field will increase the entropy, resulting in an inverse magnetocaloric effect. The equivalent reasoning also holds for hydrostatic pressure: materials for which volume increases with increasing temperature give rise to a conventional barocaloric effect (entropy decreases with application of pressure) whereas those with a decreasing volume with increasing temperature show an inverse barocaloric effect. It is also worth noticing that at constant magnetic field, materials with negative thermal expansion ( β ) will exhibit inverse barocaloric effect (equation (1)). Experimental details Ingots were prepared by arc melting the pure elements under argon atmosphere in the stoichiometric ratio. The composition was determined by energy-dispersive X-ray photoluminiscence analysis to correspond to LaFe 11.33 Co 0.47 Si 1.2 . The sample was annealed at 1,323 K for 15 days and quenched. Room temperature powder X-ray diffraction patterns were recorded using a Bruker AXS diffractometer (Cu K α radiation, 2 θ range from 20° to 80° with a step size of 0.02°). Temperature-dependent high-resolution X-ray powder diffraction measurements were performed on a transmission mode diffractometer using Debye–Scherrer geometry equipped with horizontally mounted INEL cylindrical position sensitive detectors containing 4,096 channels (0.029° 2 θ step) and by using monochromatic Cu K α radiation. Temperature was controlled by means of a liquid nitrogen 700 series Oxford Cryostem Cooler. The heating rate between the measurements was 1.3 K min −1 and, before data collection, the sample temperature was stabilized for 15 min. Magnetization measurements were carried out using a superconducting quantum interference device magnetometer. From these data, the magnetic-field-induced entropy change was numerically computed, taking into account the procedures described in (ref. 24 ), to avoid undesired overestimated values. Specific heat was measured using a modulated differential scanning calorimeter. Hydrostatic pressure calorimetry was carried out in a purpose-built calorimeter described in (ref. 7 ). From calorimetric curves at selected values of the hydrostatic pressure p , the entropy change (referenced to a given state at T 0 ) is computed as: where is the heat flux and is the heating/cooling rate. For direct adiabatic temperature measurements, a chromel–alumel thermocouple was embedded into the sample. In pressure measurements, the sample was placed into the calorimeter and it was first cooled down under applied pressure to a temperature low enough to ensure that the whole sample was in the low-temperature phase. Then, it was heated (keeping the applied pressure) up to the measuring temperature. After thermalization, the pressure was rapidly released and the output of the thermocouple was recorded at a rate of 1 Hz. This procedure was repeated for each measuring temperature. The effect of thermal losses to the surroundings was quantified by performing experiments at temperatures well above and well below the transition. For magnetic measurements, the device described in (ref. 25 ) was used. The sample was first brought to a temperature high enough to ensure that it was on the high-temperature phase. Then, it was cooled down to the desired temperature, allowed to thermalize, and magnetic field was rapidily applied (at a rate 1 T s −1 ) while the output of the thermocouple was recorded at a rate 0.5 Hz. After 30 s, the field was removed (at a rate 1 T s −1 ). This procedure was repeated for each measuring temperature. How to cite this article: Mañosa, L. et al . Inverse barocaloric effect in the giant magnetocaloric La–Fe–Si–Co compound. Nat. Commun. 2:595 doi: 10.1038/ncomms1606 (2011).